Giant negative linear compression positively coupled to massive thermal expansion in a metal–organic framework Materials with negative linear compressibility are sought for various technological applications. Such effects were reported mainly in framework materials. When heated, they typically contract in the same direction of negative linear compression. Here we show that this common inverse relationship rule does not apply to a three-dimensional metal–organic framework crystal, [Ag(ethylenediamine)]NO 3 . In this material, the direction of the largest intrinsic negative linear compression yet observed in metal–organic frameworks coincides with the strongest positive thermal expansion. In the perpendicular direction, the large linear negative thermal expansion and the strongest crystal compressibility are collinear. This seemingly irrational positive relationship of temperature and pressure effects is explained and the mechanism of coupling of compressibility with expansivity is presented. The positive coupling between compression and thermal expansion in this material enhances its piezo-mechanical response in adiabatic process, which may be used for designing new artificial composites and ultrasensitive measuring devices. Most materials are compressed in all directions by hydrostatic pressure, and only few materials exhibit negative linear/area compressibility (NLC/NAC) [1] . Such materials are coveted for piezo-responsive applications, for example, in ultrasensitive pressure detectors and robust shock-absorbing composites [2] , [3] , [4] . Till recently mainly simple inorganic systems were associated with the NLC [5] , [6] , albeit of relatively weak compressibility magnitude, as for example, of about −2.0 TPa −1 in α-cristobalite-structured BAsO 4 (ref. 7 ). The isothermal compressibility coefficient is defined as β l =−(∂ln l /∂ p ) T ; subscripts 1, 2 and 3 at β refer to the orthogonal axes of the strain tensor, whereas letters a , b and c to the crystal axes. More recently, an extensive search for materials with stronger NLC has been focused on engineering mechanistic models of ‘wine-rack’ or ‘lattice-fence’ frameworks [1] . Their elements are connected by flexible ‘hinges’ allowing the coupling of orthogonally directed NLC with positive linear compressibility (PLC). Metal–organic complex [Fe(dpp) 2 (NCS) 2 ]·py (dpp=dipyrido[3,2-a:2′3′-c]phenazine, py=pyridine) [8] and hydrogen-bonded molecular co-crystal of methanol monohydrate [9] were modelled by such hinged frameworks. In the materials of wine-rack structure the NLC and negative thermal expansion (NTE) were correlated, according to the ‘inverse relationship’ of pressure and temperature. This rule was formulated for structures of minerals built of polyhedra and it states that structural changes upon compression are similar to those upon cooling [10] . The only known exception to this rule concerns the rutile-type compounds [11] . Likewise, the collinear NTE and NLC were reported in a series of cyanide-bridged coordination polymers, such as Ag 3 [Co(CN) 6 ] (refs 12 , 13 ) and KMn[Ag(CN) 2 ] 3 (ref. 14 ). The strain along the framework layers was modelled by a wine-rack of rigid linker-ligands flexibly coordinated to Ag ‘hinges’. More recently, a remarkably strong NLC of −42(5) TPa −1 over a wide pressure range from 0.1 MPa to 1.8 GPa along the c axis of Zn[Au(CN) 2 ] 2 was explained by distortions of its β -quartz-like honeycomb framework supported by helical aurophilic interactions [15] , [16] . This impressive externally stimulated strain initiated further studies on elastic and thermal effects in soft porous metal–organic frameworks (MOFs). For example, in the wine-rack structure of MIL-47(V IV ) mechanical pressure causes large ‘breathing’, the term describing the colossal crystal-volume change of 43% between large-pore and narrow-pore phases [17] . The uptake of guest molecules strongly interacting with the host framework considerably enhances the linear responses of exceptional positive thermal expansion (PTE) coupled to NTE in Zn(II)MOF (ref. 18 ), FMOF-1 (ref. 19 ) and other porous coordination polymers [20] , [21] . Like in zeolites [22] , the NLC and negative bulk modulus (that is, the inverse of crystal-volume compression) of HKUST-1 (ref. 23 ), MOF-5 (ref. 24 ) and ZIF-8 (ref. 25 ) are caused by hydrostatic fluid (for example, small alcohol molecules) squeezed by pressure into the framework cavities. Hydrostatically compressed zeolitic imidazolate frameworks (ZIFs) are exceptionally soft due to the cooperative rearrangement of their bonds (for example, in ZnIm) [26] or amorphization (for example, ZIF-4) [27] . There are only very few reports on the intrinsic thermo-/piezo-responsive MOFs devoid of guest molecules. The intrinsic effects of NLC, β 3 (the strain-tensor eigenvalue approximately along the c axis) of −4.3(1) TPa −1 in silver(I) 2-methylimidazolate [Ag(mim)] (ref. 28 ) and β c (exactly along the crystal c axis) of −1.8(8) TPa −1 in ammonium zinc(II) formate [NH 4 ][Zn(HCOO) 3 ] (ref. 29 ) originate from distortions of their wine-rack frameworks. These structural models of the NLC/NTE strain suggest that new materials with tunable and highly responsive mechanics can be designed by combining the concepts of wine-rack framework with host–guest interactions. For example, the anions located in cavities can be H-bonded to the main framework and regulate its distortions. Such ‘inflated’ pores would be resistant to the incorporation of other guest molecules pumped by external pressure and the supported linkers would be unlikely to collapse. Herein, we report the most exceptional interplay of thermo-/piezo-mechanical effects in a simple three-dimensional (3D) MOF crystal, [Ag(en)]NO 3 (en, ethylenediamine), with pores inflated by NO 3 − anions. Its single-crystal X-ray diffraction measurements from 120 to 360 K and from ambient pressure to 3.85 GPa have revealed the largest intrinsic thermo- and piezo-mechanical response recorded so far in MOFs, to the best of our knowledge, as well as giant NLC positively coupled with large PTE, contrary to the inverse-relationship rule. Framework structure of [Ag(en)]NO 3 -I Two polymorphs of [Ag(en)]NO 3 have been known [30] , [31] . Presently, we have determined that polymorph I, denoted [Ag(en)]NO 3 -I, of monoclinic space group C 2/ c and Z =4, is stable at ambient conditions. In its structure, shown in Fig. 1 , each Ag(I) cation is planar-square fourfold coordinated by two adjacent Ag(I) cations along [001] and by two nitrogen atoms of en-ligands. Two en-ligands are attached alternatively to each Ag cation located at z =0 along direction [110] and to these at z =1/2 along direction . Thus the Ag(I) pillars are connected by these en-linkers parallel to the ab plane. The Ag˙˙˙Ag argentophilic contacts act like hinges, allowing a considerable flexibility of the 3D coordination CdSO 4 -type framework [32] . In the one-dimensional (1D) channels extending along the c axis of [Ag(en)]NO 3 -I, the nitrate NO 3 − ions are NH˙˙˙O and CH˙˙˙O hydrogen-bonded to the framework (H˙˙˙O distances of 2.383–2.693 Å at ambient conditions, cf . Fig. 1 , Supplementary Figs 1 and 2 ). 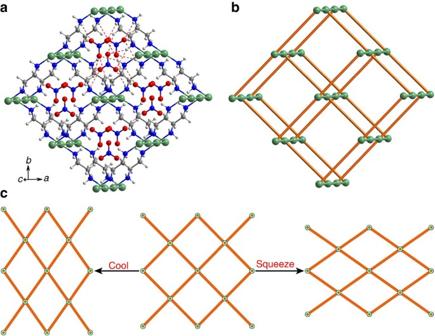Figure 1: Structure of [Ag(en)]NO3-I and its flexible coordination framework. (a) The framework of Ag+cations linked by NH2(CH2)2NH2(en) ligands viewed approximately along the channels filled with anions NO3–. The NH˙˙˙O and CH˙˙˙O hydrogen bonds are indicated as red dashed lines (cf.Supplementary Fig. 1). (b) The framework of CdSO4-type topology. (c) The schematic illustration exaggerating the ‘wine-rack’ motif responses to temperature and pressure. Colour code: green balls and sticks represent Ag˙˙˙Ag bonds, orange struts –en–Ag–en–, grey atoms C, red O, blue N, light grey H. Figure 1: Structure of [Ag(en)]NO 3 -I and its flexible coordination framework. ( a ) The framework of Ag + cations linked by NH 2 (CH 2 ) 2 NH 2 (en) ligands viewed approximately along the channels filled with anions NO 3 – . The NH˙˙˙O and CH˙˙˙O hydrogen bonds are indicated as red dashed lines ( cf . Supplementary Fig. 1 ). ( b ) The framework of CdSO 4 -type topology. ( c ) The schematic illustration exaggerating the ‘wine-rack’ motif responses to temperature and pressure. Colour code: green balls and sticks represent Ag˙˙˙Ag bonds, orange struts –en–Ag–en–, grey atoms C, red O, blue N, light grey H. Full size image Thermal expansion of [Ag(en)]NO 3 -I The crystal expansion is highly anisotropic and almost linear in all the 120−360 K range ( Fig. 2a and Supplementary Fig. 3 , Supplementary Table 1 ). The massive NTE coefficient of parameter b , α b =−89.7(15) MK −1 ( b shrinks by 2.2%), is an order of magnitude larger than that of well-known isotropic NTE material ZrW 2 O 8 (−9.1 MK −1 ) [33] , about four times larger than those of two other CdSO 4 -type MOFs, [Ag(mim)] (−24.5(8) MK −1 ) [28] and HMOF-1 (−21(3) MK −1 ) [34] , comparable to those of recently reported MCF-34 (ref. 21 ) and fu-MOFs [35] , but ~73% of the colossal values of cyanide-based inorganic material Ag 3 [Co(CN) 6 ] (−126(4) MK −1 ) [13] and half of that in molecular organic crystal ( S , S )-octa-3,5-diyn-2,7-diol (−190(25) MK −1 ) [36] ( Supplementary Tables 2 and 3 ). In [Ag(en)]NO 3 -I the massive NTE along b is coupled through the hinged-framework structure to the colossal PTE, the strain eigenvector of which is approximately parallel to the direction, inclined by 24.2° to axis a ( Supplementary Fig. 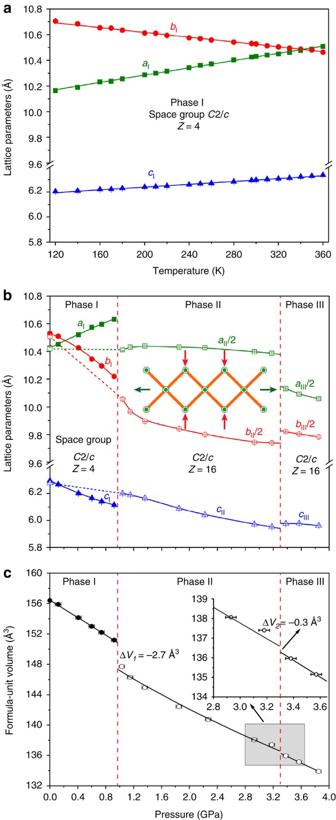Figure 2: Temperature and pressure dependence of lattice parameters in [Ag(en)]NO3. (a) The thermal expansion of phase I:a(green squares),b(red circles) andc(blue triangles). (b) Unit-cell dimensions change during hydrostatic compression of phases I–III. The lattice parameters of phase II at 0.1 MPa/293 K (ref.31) have been included for comparison and they have been connected to high-pressure data of phase II by red, blue and green dotted lines. (c) The third- and second-order Birch–Murnaghan (phases I and II) and linear (phase III) fits to the formula-unit volume (V/Z) data. These equations of state have been used for calculating the ΔVdrop at transitions between phases I/II and between phases II/III, enhanced in the inset. The inset inbconnects the framework distortions with the unit-cell dimensions (cf.Fig. 1). The phase transitions at 0.97 and 3.30 GPa are indicated by vertical red dashed lines inbandc. 4 and Supplementary Table 2 ). The corresponding mean eigenvalue, α 3 of +149.2(12) MK −1 is comparable to the large thermal response of +144(9) MK −1 in Ag 3 [Co(CN) 6 ] (ref. 13 ). The volume thermal-expansion coefficient α V of [Ag(en)]NO 3 -I, equal to 95.8(20) MK −1 , is three times larger than those of conventional engineering materials (for example, steel, 35 MK −1 ) [37] . Figure 2: Temperature and pressure dependence of lattice parameters in [Ag(en)]NO 3 . ( a ) The thermal expansion of phase I: a (green squares), b (red circles) and c (blue triangles). ( b ) Unit-cell dimensions change during hydrostatic compression of phases I–III. The lattice parameters of phase II at 0.1 MPa/293 K (ref. 31 ) have been included for comparison and they have been connected to high-pressure data of phase II by red, blue and green dotted lines. ( c ) The third- and second-order Birch–Murnaghan (phases I and II) and linear (phase III) fits to the formula-unit volume ( V / Z ) data. These equations of state have been used for calculating the Δ V drop at transitions between phases I/II and between phases II/III, enhanced in the inset. The inset in b connects the framework distortions with the unit-cell dimensions ( cf . Fig. 1 ). The phase transitions at 0.97 and 3.30 GPa are indicated by vertical red dashed lines in b and c . Full size image Compression of [Ag(en)]NO 3 -I High-pressure single-crystal X-ray diffraction measurements of [Ag(en)]NO 3 were performed with a modified Merrill–Bassett diamond-anvil cell (DAC). We chose isopropanol as a hydrostatic pressure-transmitting medium [38] and pressure was calibrated by ruby-fluorescence [39] . The most striking giant NLC along axis a continues monotonically to 0.97 GPa. This pressure induces a discontinuous transition to phase II, [Ag(en)]NO 3 -II, previously determined as a metastable polymorph at ambient pressure [31] , and 3.30 GPa induces another discontinuous transition to a new phase III, [Ag(en)]NO 3 -III ( Fig. 2 and Supplementary Tables 4 and 5 ). The NLC of [Ag(en)]NO 3 -I is very strong and its strain tensor eigenvector β 3 of −28.4(18) TPa −1 is inclined by 24.2° to the a axis and perpendicular to axis b ( Supplementary Fig. 4 and Supplementary Table 6 ). Thus the orientation of axes of the thermal-expansion and hydrostatic compression strain tensors is nearly the same ( Supplementary Fig. 4 ). The NLC β 3 magnitude is comparable to those in the most extreme NLC inorganic materials, such as Ag 3 [Co(CN) 6 ] phase I stable to 0.19 GPa (average β c =−76(9) TPa −1 ) [12] and phase I of Zn[Au(CN) 2 ] 2 , stable to 1.8 GPa (average β c =−42(5) TPa −1 ) [15] . To the best of our knowledge, compound [Ag(en)]NO 3 -I shows the strongest NLC yet observed in MOFs ( Supplementary Table 7 ). The strongest PLC in [Ag(en)]NO 3 -I is along axis b and the corresponding coefficient β b equals 39.1(21) TPa −1 . The third-order Birch–Murnaghan equation of state gives the zero-pressure bulk modulus B 0 of 27.5(16) GPa, and its pressure derivative B ′ of −1.6(31) indicates that the material becomes increasingly softer under pressure ( Supplementary Table 8 and Supplementary Methods ). Such a pressure-induced softening was observed also in other framework materials, that is, Zn[Au(CN) 2 ] 2 (ref. 15 ) and Zn(CN) 2 (refs 40 , 41 ). Phase transitions and compression of phases II and III The transition at 0.97 GPa to phase II retains the space group C 2/ c and the crystal directions, but the lattice main translations extend to the 2 × 2 × 1 supercell with Z increased fourfold to 16 ( Figs 2b and 3 and Supplementary Fig. 5 ). The framework of [Ag(en)]NO 3 -II preserves the CdSO 4 -topology ( Supplementary Fig. 6 ). At the transition, the formula-unit volume ( V / Z ) drops by 2.7 Å 3 ( Fig. 2c ). At 0.1 MPa, phase II is more dense than phase I (2.460 versus 2.442 g cm −3 ) [31] . In our experiments on releasing pressure, phase II transformed back to phase I, which confirms that polymorph II is metastable at 0.1 MPa (see Supplementary Methods ). 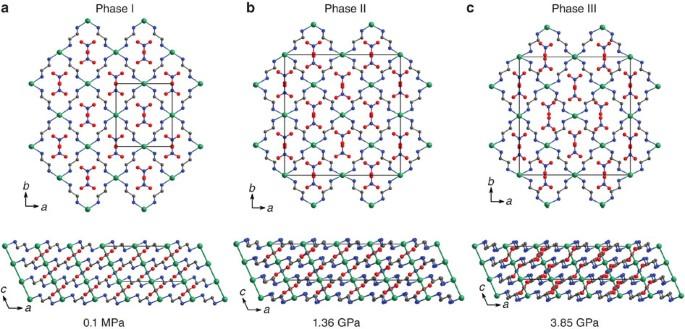Figure 3: Structural relationships among [Ag(en)]NO3phases I–III. The crystal structure viewed along the [001] and [010] directions. (a) Phase I at ambient pressure. (b) Phase II at 1.36 GPa. (c) Phase III at 3.85 GPa. The unit-cell parameters of phase I is doubled along axesaandbin phases II and III. Atoms coloured as inFig. 1. Figure 3: Structural relationships among [Ag(en)]NO 3 phases I–III. The crystal structure viewed along the [001] and [010] directions. ( a ) Phase I at ambient pressure. ( b ) Phase II at 1.36 GPa. ( c ) Phase III at 3.85 GPa. The unit-cell parameters of phase I is doubled along axes a and b in phases II and III. Atoms coloured as in Fig. 1 . Full size image Most remarkably, despite the discontinuous transition, the NLC of phase I persists in phase II till 1.5 GPa. The corresponding eigenvector of the strain tensor is inclined by 13° to the a axis and the NLC coefficient β 3 is equal −9.3(8) TPa −1 ( Supplementary Table 9 ). The hinged-framework structure of [Ag(en)]NO 3 -II implies that this NLC is coupled to the PLC along axis b . On approaching 1.5 GPa this relation becomes considerably weaker and the NLC along axis a levels off and the compression becomes positive along this direction at still higher pressure ( Fig. 2b ). Although the NLC effect between 0.97 and 1.5 GPa is weaker than in phase I, it is still stronger than that observed in MOFs [Ag(mim)] (ref. 28 ) and [NH 4 ][Zn(HCOO) 3 ] (ref. 29 ). The unit-cell volume can be well fitted by the second-order Birch–Murnaghan equation of state in the 0.97 to 3.18 GPa range; the bulk modulus B 0 of 22.7(11) GPa and B ′ of 4 show that phase II is somewhat softer than phase I ( Supplementary Table 8 , Supplementary Methods ).The volume compression of phase II is monotonic despite the reversed linear compression along axis a above 1.5 GPa ( Fig. 2c ). At 3.30 GPa, on the transition to [Ag(en)]NO 3 -III, parameter a is reduced by 1.85%, while b and c expand by 0.83 and 0.40%, respectively ( Fig. 2b and Supplementary Table 5 ). This discontinuous strain relation between reduced a and increased b is also consistent with the wine-rack distortion mechanism. At the transition, a highly anisotropic discontinuous NAC is approximately parallel to the bc plane; the β angle abruptly decreases by about 0.26° ( Supplementary Fig. 7 ) and the formula-unit volume collapses by ~ 0.3 Å 3 ( Fig. 2c ). The transition between phases II and III is isostructural because the lattice nodes and the space group are not changed. It is also characteristic of isostructural transitions that they are discontinuous [42] . Despite its isostructural character, the transition significantly changes elastic properties of the crystal: the least compressible in phase II parameter a becomes the softest of all parameters in phase III ( Fig. 2b and Supplementary Table 10 ). Starting from ~0.20 GPa the length of en-linkers is markedly compressed and in phase III it considerably contributes to breaking the wine-rack coupling between axes a and b . Consequently, within phase III all directions are compressed, at least up to the experimental limit of 3.85 GPa. The intrinsic mechanical response of [Ag(en)]NO 3 -I is much stronger than that in MOFs of similar CdSO 4 -topology, [Ag(mim)] (ref. 28 ) and HMOF-1 (ref. 34 ). This exceptional NTE/NLC of [Ag(en)]NO 3 -I arises from several factors. The mechanical response of framework materials depends on their topology, organic linkers and even the guest molecules inside the voids. Although both [Ag(en)]NO 3 -I and Ag(mim) have the same CdSO 4 wine-rack topology and the en and min linkers are relatively rigid, their frameworks are substantially different. These frameworks differ by the charges of the linkers, as the en linker is neutral and min is anionic, and in the structure and directions of Ag–N coordination bonds, parallel in [Ag(en)]NO 3 -I and forming the subtended angle of 145° in Ag(min). The linkers in Ag(min) are free to rotate, whereas in [Ag(en)]NO 3 -I they are H-bonded to NO 3 groups; there are hardly any voids in Ag(min) and they are large filled voids in [Ag(en)]NO 3 -I. Most importantly, the positions of NO 3 – anions in [Ag(en)]NO 3 -I are coupled by directional NH˙˙˙O hydrogen bonds to the linkers and the strain in the structure is transmitted to other directions through the anions. There are also numerous weaker CH˙˙˙O hydrogen bonds between the framework and the anions. The soft argentophilic Ag˙˙˙Ag bonds, acting as hinge pins, combine the zigzag-like en-ligand struts into the 3D supramolecular network. The Ag atoms occupy the inversion centres, and the framework distortions, in response to temperature and pressure, are directly reflected in the lattice parameters. The lattice-framework relations in [Ag(en)]NO 3 -I can be expressed as formulas: where θ is the hinge angle equal to arctan( a / b ), r is the Ag˙˙˙Ag distance along one en linker and d (Ag˙˙˙Ag) is the Ag˙˙˙Ag bond length along axis c ( Fig. 4a,b ). Analogous formula are valid for phases II and III, but there the a and b unit-cell parameters (doubled) are equal to 4 r sin θ and 4 r cos θ , respectively ( cf . Fig. 3 ). 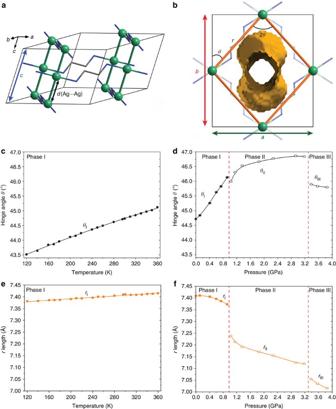Figure 4: The thermo- and piezo-mechanical response of [Ag(en)]NO3. (a) Perspective view of framework of phase I. (b) The framework projected down axisc. Unit cells of phases II and III are doubled along axesaandb, but the framework structure is preserved. One void in the structure at 0.1 MPa/296 K is shown for a probing sphere 1.2 Å in radius moved in 0.2 Å steps, after removing the NO3–anions. (c) The temperature dependence of hinge angleθ(black circles). (d) Hinge angleθchanges in hydrostatically compressed phases I (full circles), II and III (open circles). (e) Lengthrof strut along the en-linkers in theabplane in phase I (orange squares). (f) Evolution of strutrlength in phases I (full squares), II and III (open squares) under compression. The estimated s.d. values are smaller than the plotted symbols. Figure 4: The thermo- and piezo-mechanical response of [Ag(en)]NO 3 . ( a ) Perspective view of framework of phase I. ( b ) The framework projected down axis c . Unit cells of phases II and III are doubled along axes a and b , but the framework structure is preserved. One void in the structure at 0.1 MPa/296 K is shown for a probing sphere 1.2 Å in radius moved in 0.2 Å steps, after removing the NO 3 – anions. ( c ) The temperature dependence of hinge angle θ (black circles). ( d ) Hinge angle θ changes in hydrostatically compressed phases I (full circles), II and III (open circles). ( e ) Length r of strut along the en-linkers in the ab plane in phase I (orange squares). ( f ) Evolution of strut r length in phases I (full squares), II and III (open squares) under compression. The estimated s.d. values are smaller than the plotted symbols. Full size image The general empirical evidence reported so far mainly for minerals [10] , but also for framework materials [12] , [15] , MOFs [28] , as well as organic compounds [9] , [43] , [44] , show that in most compounds temperature and pressure cause the opposite strain, that is, the NLC exists in the direction of NTE or of the smallest PTE. This common behaviour is known as the inverse relationship rule [10] . The thermal expansion and compression presently reported for [Ag(en)]NO 3 -I violate this rule ( Supplementary Fig. 8 ). Between 120 and 360 K the hinge angle θ increases by 1.60° ( Fig. 4c ), a expands by 0.34 Å and b contracts by 0.24 Å ( Fig. 2a ). This θ ( T ) increase exactly correlates with the colossal PTE along a and NTE along b , according to equations (1) and (2). Pressure increases the θ hinge angle most significantly through phase I (by 1.42° to 0.92 GPa), it slightly drops by ~0.1° at the transition to phase II, but then continues to rise through phase II up to 3.30 GPa by another 0.85°. This framework distortion generates the NLC of [Ag(en)]NO 3 -II up to ~1.5 GPa, when the compression of parameter r , comprising the coordination bonds Ag–N and of the en-linkers ( Fig. 4 ), is sufficiently high to counteract the NLC effect generated by increasing θ . Equations (1) and (2) of the wine-rack model continue to exactly describe the unit-cell parameters, but above 0.97 GPa the changes of r ( P ) significantly contribute to the [Ag(en)]NO 3 compression. The external stimuli also induce more subtle, but equally intriguing, systematic responses in the [Ag(en)]NO 3 -I structure. For example, the Ag1−N1 bonds lengthen with increasing pressure and their initial increase with temperature stops at ~300 K, above which they slightly decrease with temperature ( Supplementary Fig. 9 and Supplementary Tables 11 and 12 ). There are no apparent changes in the conformation of en-ligands in all [Ag(en)]NO 3 structures investigated at increased temperature and pressure, which is consistent with s - trans molecular conformation (that is, the torsion angle of N−C−C−N is equal to 180°) in all three polymorphs of neat ethylenediamine (en) at various temperature and pressure conditions [44] . The violation of the inverse-relationship rule by [Ag(en)]NO 3 -I indicates that the modus operandi of this fascinating highly efficient elastic sensor cannot be rationalized by its wine-rack framework alone. The colossal strain in [Ag(en)]NO 3 -I arises from the interplay of flexible MOF with thermally regulated dynamics of NO 3 – anions and en-linkers through a tailored network of NH···O and CH˙˙˙O hydrogen bonds. The H-bonds and frameworks were so far used separately as the most basic elements in engineering crystal of required properties. The small and ovoid NO 3 − anions are sensitive to temperature and pressure and parameters describing their positions, orientations and hydrogen bonds monotonically change from 0.1 MPa to 0.92 GPa, and from 360 to 120 K ( Supplementary Figs 10 and 11 ). Although the effect of temperature is considerably smaller than that of pressure, the shifts of NO 3 groups comply with the inverse relationship rule. The NO 3 group orientation described by the dihedral angle φ 2 relative to the ab plane increases by ~1.3° from 120 to 360 K, while it is reduced by −3.0° within pressure range of phase I ( Supplementary Fig. 10 ). The dihedral angles of the en ligand and of NO 3 – anions with the ab plane in phase II are comparable to those in phase I. However, all the dihedral angles abruptly increase above 3.30 GPa in phase III. The dihedral angle φ 1 between en-ligands and the ab plane is increased by 5.8° between 120 to 360 K, while it is reduced by 13.2° at 0.92 GPa ( Supplementary Fig. 10 ). Thus, changes of all these dimensions obey the inverse relationship rule. The violation of the inverse relationship rule in [Ag(en)]NO 3 -I results from the interactions of NO 3 − anions with the framework, as described below. In [Ag(en)]NO 3 -I the NO 3 − anions are located in the channel voids of elliptic cross-section significantly elongated along the direction of axis b . It is essential for the elastic properties of [Ag(en)]NO 3 -I that this elongation of the cross-section of voids is due to the position of en-linkers, whereas the hinge angle 2 θ directly describes the mutual directions of the struts and not the shape of voids. Thus, despite the 2 θ opening close to 90° at normal conditions, the cross-section of voids is significantly elongated, as illustrated in Fig. 4b . The NO 3 − anions can be more efficiently contained in the channel voids, when their cross-section becomes more rounded. Increased temperature easily activates vibrations of the small ovoid and weakly bonded in this structure NO 3 − anions. Their vibrations require more space and ‘inflate’ the voids. Hence their more rounded cross-section, which is possible when the framework distortions consistent with the lattice expansion along a and contraction along b are generated. Thus, the increased ‘internal pressure’ in the voids is partly relieved by the expansion of the crystal along a and its contraction along b , in accordance with the wine-rack distortion. This void-shape change, which can be clearly observed visually ( Supplementary Fig. 12a ), results in the void volume increasing by 13.8% between 120 and 360 K. According to the inverse relationship rule, one would expect that at increased pressure the framework would close up to compress the voids. However, [Ag(en)]NO 3 -I responses to pressure differently than expected, owing to the combination of inherent features of the framework with the shape of filled voids. In the compressed framework the en-linkers decrease their inclination to plane ab , at the rate plotted in Supplementary Fig. 10b . By protruding more toward the voids, the en-linkers make the cross-section of the voids narrower along a . In turn, this narrowing additionally (apart of the framework struts compression, r ( P ) plotted in Fig. 4f ) reduces the volume of the voids. Thus at high pressure, the voids become even less rounded, primarily due to the rotation of en-ligands ( Supplementary Fig. 12b ). This effect of en-ligands rotations and voids narrowing is partly counteracted by the hinge-angle θ opening, and the overall voids-volume reduction is 12.6% between 0.1 MPa and 0.92 GPa. The θ increase in response to the voids narrowing along the a direction (see Supplementary Fig. 12b ) can be illustrated by the scissors-like opening of the struts, pushed apart by the voids contents (NO 3 – anions). The θ -angle increase ( Fig. 4 ), in turn, results in the NLC along the a axis and PLC along axis b . In order to better understand this effect of pressure, we have hypothetically considered the opposite direction of the framework distortion, that is, ‘scissors-closing’ of struts and the θ angle reduction. It would have caused, in conjunction with the rotations of en-linkers, a more significant narrowing of the voids and, in consequence, even a more significant voids-volume reduction than this observed. We have estimated that the voids volume would be reduced by 19% at least. Thus, the observed distortion of the framework counteracts such a strong collapse of voids, because they are filled with NO 3 − anions. It is remarkable that the effects of ‘voids-rounding’ at higher temperature and ‘scissors-opening’ of struts in increased pressure act in the same direction. Hence, the positive coupling between the [Ag(en)]NO 3 -I crystal expansivity and compressibility. In phase II these effects, of the en-linkers inclination changes and the rounding reaction of voids accommodating ovoid NO 3 groups, prevail until 1.5 GPa (the NLC region). At still higher pressure the PLC behaviour along direction a is enforced due to the considerable compression of the framework r dimension ( Fig. 4f ). Above 1.5 GPa (in phases II) the r compression causes a secondary effect of the voids-volume reduction, which is counteracted by increased θ angle allowing a slower reduction of the volume accommodating the NO 3 groups. In summary, the direct (as opposed to inverse) relationship of temperature and pressure giant effects of PTE and NLC approximately along the a axis, coupled to NTE and PLC along axis b , has been observed in [Ag(en)]NO 3 -I. To the best of our knowledge, this is the first example of a material exhibiting such a giant anisotropic strain in response to temperature and pressure changes. These unique properties of [Ag(en)]NO 3 -I result from an interplay of several effects involving the flexible framework and its en-struts H-bonded to NO 3 – anions in its voids. High temperature increases the NO 3 – anions dynamics, and their intensified interactions with the framework around enforce the more rounded cross-section of voids, expanding along a . At high pressure the same direction of expansion is caused by the ‘scissors-like’ distortion of the framework counteracting the rotations of the struts hydrogen-bonded to the NO 3 − anions. These effects of the voids ‘inflating’ and the framework ‘scissors-opening’ in [Ag(en)]NO 3 -I account for its positive strain relation of temperature and pressure, respectively. This understanding of the structural mechanism facilitates further search for other materials with positively coupled giant NLC and PTE. Noteworthly, owing to the direct relationship of colossal temperature and pressure effects in [Ag(en)]NO 3 -I, its response to compression and adiabatic warming is enhanced. In most materials the compression and expansion partly compensate at adiabatic transformations. To our knowledge the opposite direction of this adiabatic correction was never considered. Thus, an adiabatically compressed solid warms up, which causes some expansion counteracting the compression effect by few per cent. The adiabatic compression of [Ag(en)]NO 3 -I causes along direction b an additional compression and along direction a an additional expansion, in both cases of few per cent for the compression to 0.97 GPa. This remarkable thermo-/piezo-mechanical response of [Ag(en)]NO 3 -I can be applied in thermo-mechanical sensors and second-generation pressure devices. This is a new approach for controlling the hinge movement of the host framework by anions contained in the porous channel and linked by hydrogen bonds. Such a MOF stuffing can be applied for other framework types for developing new functional hybrid materials with exceptional properties. Synthesis Single crystals of [Ag(en)]NO 3 -I were synthesized as reported previously [30] . AgNO 3 (57.9 mg, 0.34 mmol) was dissolved in 5 ml acetonitrile solution and layered carefully on top of the 5 ml o -xylene solution of ethylenediamine (20.5 mg, 0.34 mmol). Light-yellow single-crystal plates suitable for X-ray diffraction studies were obtained after 2 weeks. Single-crystal X-ray diffraction Variable temperature diffraction measurements were performed on Oxford Diffraction Xcalibur Eos (MoKα radiation, λ =0.71073 Å) diffractometer fitted with an Oxford Cryosystems cryostream in the range of 120–360 K. A single crystal (0.32 × 0.08 × 0.06 mm) was mounted on a glass fibre and glued with nail varnish. The data were initially collected at 300 K and then a series of data sets were recorded at intervals of 20 K steps down to 120 K. In the heating run, the unit-cell dimensions and diffraction data were measured at 170, 210, 250, 296, 300, 320, 340 and 360 K. Then temperature was decreased back to 350, 330, 310 and finally 300 K. The changes in the structural parameters of [Ag(en)]NO 3 -I observed in the temperature range investigated (120–360 K) are fully reversible. Data reduction and absorption correction were performed in CrysAlisPro software. The crystal structure of [Ag(en)]NO 3 -I was solved by direct methods or from the starting model of the structure at ambient conditions [30] . The structure refinement was performed by programme SHELXL-97 (ref. 45 ) for all the variable temperature crystal data ( Supplementary Table 1 and Supplementary Data 1 ). High-pressure X-ray diffraction data were measured on an Oxford Diffraction Xcalibur Eos diffractometer, with graphite-monochromated MoKα ( λ =0.71073 Å) radiation, for two single crystals mounted in two modified Merrill–Bassett DACs. Diamond anvils had culets 800 μm in diameter. The gaskets were made of tungsten foil 0.30 mm thick, with the spark-eroded hole initially 0.45 mm in diameter. Pressure was calibrated with a Photon Control spectrometer with enhanced resolution to ~3,000 pixels per 30 nm dispersion by ruby fluorescence [39] , with a precision of 0.04 GPa. The uncertainty was reduced by repeating pressure measurements before and after each diffraction-data collection. Anhydrous isopropanol [38] was used as the pressure-transmitting medium. The high-pressure diffraction data were collected between 0.12 and 3.85 GPa at 15 different pressure points ( Supplementary Tables 4 and 5 , Supplementary Methods and Supplementary Data 2 ). The centring of the DAC was performed by the gasket-shadowing method [46] . CrysAlisPro software was used for the data collection and the preliminary reduction of the data. After the intensities were corrected for the effects of DAC absorption, sample shadowing by the gasket and the sample absorption, the diamond reflections were eliminated [47] . The crystal structure of [Ag(en)]NO 3 -I at ambient condition was used as a starting model for structure refinement on high-pressure data by programme SHELXL-97 (ref. 45 ). With the aim to compare the crystal structure of phase II with phase I along the same orientation, a new lattice vector a was chosen, the transformation matrix (1 0 2 0 −1 0 0 0 −1) was utilized for the high-pressure crystal data of phases II and III. And their structure was solved by direct methods based on the previous structure at ambient conditions [31] . According to the data refinement of phases I, II and III, the en-ligands and nitrate ions were constrained to the ideal geometries and all en-ligands in phases II and III were constrained to the planar conformation. All the Ag−N distances were refined freely and the silver atoms were refined anistropically. The anisotropic values of few carbon, oxygen and nitrogen atoms were restrained to approximate isotropic shape by using command ISOR 0.05 of SHELXL-97 (ref. 45 ) The H-atoms were located from the molecular geometry, with the N−H distances equal to 0.90 Å (−NH 2 group) and 0.97 Å (−CH 2 group), and the isotropic displacement parameters 1.2 times U eq of their carriers. Calculations The coefficients of linear thermal expansion α l =(1/ l ) (∂ l /∂ T ) p (MK −1 , × 10 −6 K −1 ) and linear compressibility β l =–(1/ l ) (∂ l /∂ p ) T (TPa −1 , × 10 −3 GPa −1 ) and bulk modulus B of [Ag(en)]NO 3 were calculated by PASCal [48] . Voids calculations were performed using Mercury with the probe radius and grid spacing of 1.2 Å and 0.2 Å, respectively [49] . Accession Codes. Crystallographic data for structures reported in this paper have been deposited in the Cambridge Crystallographic Data Center under reference numbers CCDC 975792−975819 and 978930−978935. These data can be obtained free of charge via www.ccdc.cam.ac.uk/data_request/cif . How to cite this article: Cai, W. & Katrusiak, A. Giant negative linear compression positively coupled to massive thermal expansion in a metal-organic framework. Nat. Commun. 5:4337 doi: 10.1038/ncomms5337 (2014).